Naphthol radical couplings determine structural features and enantiomeric excess of dalesconols inDaldinia eschscholzii Understanding how simple molecules are pieced together in organisms may aid biotechnological manipulation and synthetic approaches to complex natural products. The mantis-associated fungus Daldinia eschscholzii IFB-TL01 produces the unusually structured immunosuppressants (±)-dalesconols A and B, along with their congener (±)-dalesconol C, with the (−)-enantiomers in excess. Here we report that these structural and stereochemical peculiarities of dalesconols A–C are a result of promiscuous and atropselective couplings of radicals derived from 1,3,6,8-tetrahydroxynaphthalene, 1,3,8-trihydroxynaphthalene and 1,8-dihydroxynaphthalene. The observed (−)-enantiomeric excess is found to depend on the dominance of particular conformers of naphthol dimer intermediates, which are ligands of laccase. Natural products facilitate the discovery of new pharmaceuticals, nutraceuticals and agrochemicals while serving as 'challenging molecules' to drive methodological innovation in organic synthesis and synthetic biology [1] , [2] . Most organisms produce chiral secondary metabolites in an optically pure form where the chirality is a key determinant in the chemistry and biology of the compounds [3] , [4] . However, the racemerization of natural asymmetric molecules and/or epimerization of a particular chiral carbon occurs in some organisms, and the processes leading to their formation are poorly understood. Some organisms generate stereoisomers in equal amounts, or with an enantiomeric excess (e.e.). This is particularly apparent in (±)-dalesconols A ( 1 ) and B ( 2 ), immunosuppressive polyketides with an unusual carbon skeleton, isolated from the culture of an ascomycete D. eschscholzii IFB-TL01 habituating originally in the Tenodora aridifolia gut [5] . Moreover, chiral high-performance liquid chromatography resolutions of (±)- 1 and (±)- 2 quantitatively collected from the fermented medium demonstrated that the fungus produced both polyketides uniformly with (−)-e.e. ( ca . 67%, see Supplementary Figs S15 and S17 in ref. 5 ). Similar results have also been observed for dalesconol C ( 3 ), a congener of this type of polyketide obtained from the regrown material of the fungus [6] . The total synthesis of the two complex and bioactive compounds has been achieved in Snyder's group [7] in 24 steps (the longest linear sequence consisting of 14 steps), and the overall yields for 1 and 2 were 1.3% and 5.2%, respectively. This was followed by the construction of the dalesconol framework [8] . Both syntheses inevitably involved toxic and costly chemicals [7] , [8] . Fermentation allowed the production of dalesconols A and B: compounds 1 (100 mg) and 2 (70 mg) were recoverable from the cell-free broth after feeding the wild-type fungal strain with malt extract (ME) (2 kg), sucrose (2 kg), and peptone (100 g) [5] . Hence, fungal fermentation may be the prefered choice for supplying the immunosuppressive polyketides. Basic knowledge of the biosynthesis of the dalesconols may improve the fungal production of these compounds. Though hampered initially by the genetic obscurity of the producing fungus, we were motivated to address the biosynthetic aspects governing the generation of the unique carbon skeleton and substitution pattern as well as the (−)-e.e. characteristic of those polyketides. Surprisingly, the unusual framework and oxygenation pattern of polyketides 1 – 3 are afforded by the promiscuous couplings of different naphthol radicals ( Fig. 1 ). The (−)-e.e. was computed to depend on the conformational dominance of the naphthol dimer radicals as laccase substrates, which allows the (–)-stereoisomer overgeneration. This knowledge concerning the C–C bond formation via phenoxy radical couplings may inspire the manipulation of dalesconol microbial production and synthetic variants of the phenolic compounds. 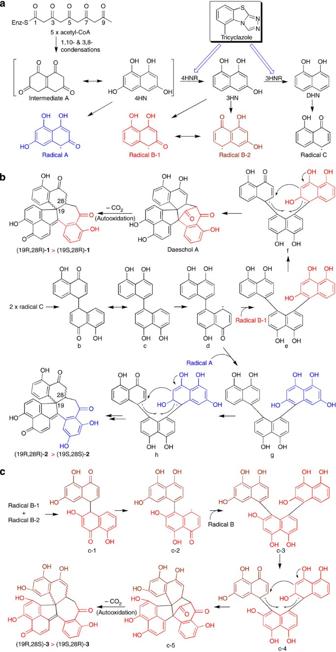Figure 1: Promiscuous couplings of naphthol radicals to form dalesconols A–C (1–3). (a) 4HN is the common precursor of naphthol radicals A, B-1 (interchangeable with B-2) and C. Tricyclazole is an inhibitor of the 4HNR and 3HNR with greater affinity for the latter. (b) Dalesconols A–B (1–2) are formed through the coupling of radicals A, B-1 and C, and (c) dalesconol C (3) through that of radicals B-1 and B-2. Figure 1: Promiscuous couplings of naphthol radicals to form dalesconols A–C (1–3). ( a ) 4HN is the common precursor of naphthol radicals A, B-1 (interchangeable with B-2) and C. Tricyclazole is an inhibitor of the 4HNR and 3HNR with greater affinity for the latter. ( b ) Dalesconols A–B ( 1 – 2 ) are formed through the coupling of radicals A, B-1 and C, and ( c ) dalesconol C ( 3 ) through that of radicals B-1 and B-2. Full size image Confirmation of naphthol residues as building blocks Scrutinizing the aromatization and substitution patterns of dalesconols A–C ( 1 – 3 ), we hypothesized that they could be biosynthetically constructed via a combination of three naphthol residues with a carbon eliminated through an autooxidation reaction we witnessed recently [6] . This assumption was substantiated by the fact that the fungus produced as well naphthol-dimerized derivatives such as dihydrosphaerolone and 2,16-dihydroxyl-benzo[ j ]fluoranthene (a new potent immunosuppressor) [5] , [6] . To confirm this prediction, we searched for the genetic evidence to lead to the identification of pksTL , a gene encoding 1,3,6,8-tetrahydroxynaphthalene synthase (4HNS). This enzyme has been demonstrated to be highly conserved in ascomycetous fungi [9] , allowing thereby the design to degenerate PCR primers, with which the partial sequence of pksTL ( ∼ 3,102 bp) was cloned. This observation was reinforced by the whole 7,565-bp gene ascertained using a genome-mining strategy (GenBank Nucleotide Core accession code: HM545254 ). The deduced amino-acid sequence of polyketide synthase encoded by pksTL gene (PKSTL) showed a high homology to those from Nodulisporium sp. PKS1 (ref. 10 ), Xylaria sp. PKS12 (ref. 11 ) and Colletotrchum lagenarium PKS1 (ref. 12 ). Moreover, PKSTL was analyzed by SEARCHPK [13] , disclosing the presence of five domains (all conserved in the PKS family) consisting of ketosynthase (KS, 384–822), acyltransferase (AT, 918–1209) and two acyl carrier proteins (ACP, 1672–1730 and 1785–1867), thioesterase–claisen cyclase (TE/CLC, 1930–2157). To explore the function of the pksTL gene, the effects of its disruption on the fungus were investigated subsequently to obtain an albino mutant, which was demonstrated to be weaker in viability and pigmentation, and unable to generate any of the polyketides 1 – 3 and dihydrosphaerolone (a naphthol dimer) as indicated by the liquid chromatography - tandem mass spectrometry (LC-MS/MS) analysis ( Fig. 2b , Supplementary Fig. S1 ). This observation indicates that the pksTL gene of D. eschscholzii , containing the five domains governing, respectively, KS, AT, ACP, ACP and TE/CLC, participates in the biosynthesis of these naphthol-derived polyketides ( Fig. 2a ). 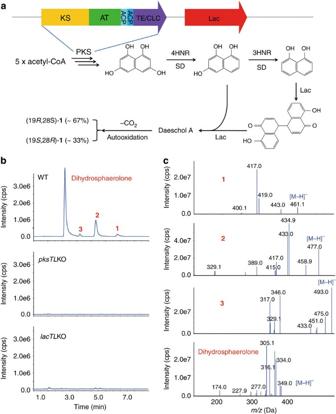Figure 2: Genetic evidence supportive of the proposed biosynthetic pathways of dalesconols A–C (1–3). (a) Exemplified by1, the catalytic reaction was mediated by an iterative PKS and necessary proteins whose sequence scales were represented approximately. Lac, laccase; SD, scytalone dehydratase. (b,c) Comparisons of LC–MS/MS profiles in an EIC (extracted ion chromatogram) mode of wild-type (WT),pksTLgene knockout (pksTLKO) andlacTLgene knockout (lacTLKO) strains ofD. eschscholzii, the latter two being unable to produce1–3and dihydrosphaerolone (a naphthol dimer). In the on-line electrospray ionization interface (ESI)–MS spectra of1–3and dihydrosphaerolone recorded in negative-ion mode, the chosen characteristic parent/daughter ion pairs were: 461.0>443.0 (1), 477.0>435.0 (2), 493.0>346 (3) and 349>277 (dihydrosphaerolone), which were acquired in MRM (multiple reaction monitoring) mode. Figure 2: Genetic evidence supportive of the proposed biosynthetic pathways of dalesconols A–C (1–3). ( a ) Exemplified by 1 , the catalytic reaction was mediated by an iterative PKS and necessary proteins whose sequence scales were represented approximately. Lac, laccase; SD, scytalone dehydratase. ( b , c ) Comparisons of LC–MS/MS profiles in an EIC (extracted ion chromatogram) mode of wild-type (WT), pksTL gene knockout ( pksTL KO) and lacTL gene knockout ( lacTL KO) strains of D. eschscholzii , the latter two being unable to produce 1 – 3 and dihydrosphaerolone (a naphthol dimer). In the on-line electrospray ionization interface (ESI)–MS spectra of 1 – 3 and dihydrosphaerolone recorded in negative-ion mode, the chosen characteristic parent/daughter ion pairs were: 461.0>443.0 ( 1 ), 477.0>435.0 ( 2 ), 493.0>346 ( 3 ) and 349>277 (dihydrosphaerolone), which were acquired in MRM (multiple reaction monitoring) mode. Full size image As described [14] , 4HN can be transformed in most fungi into 3HN and 1,8-dihydroxynaphthalene (DHN) under tandem catalyses of 4HN reductase (4HNR), 3HN reductases (3HNR) and scytalone dehydratase ( Fig. 2a ). Accordingly, we presumed that polyketides 1 – 3 could have been produced by promiscuous coupling of 4HN, 3HN and DHN motifs ( Fig. 1b,c ). This hypothesis was confirmed by the identification of 3HNR-, 4HNR- and scytalone dehydratase-encoding genes (GenBank Nucleotide Core accession codes: JX025155 , JX025154 and JX025156 ) by genome mining from separate gene clusters, and by the inhibition test with tricyclazole, a specific co-inhibitor of 4HNR and 3HNR [14] , whose presence in the medium should substantially deviate the fungal synthesis of 1 – 3 . As determined by the LC-MS/MS approach, the production of 1 and 2 was shown remarkably reduced in the batches treated with tricyclazole at 30 and 50 mg l −1 , and both failed to be detected upon the fungal exposure to tricyclazole at 100 mg l −1 . But dalesconol C ( 3 ) remained detectable in these treatments, suggesting that its production was independent of DHN ( Fig. 3 ). Moreover, if grown with tricyclazole at 150 mg l −1 in the same medium, none of the polyketides 1 – 3 could be detected in the fungal culture. Moreover, dihydrosphaerolone derived from scytalone and 3HN [15] was detectable in the tricyclazole-treated batches, but decreased as the tricyclazole concentration increased ( Supplementary Fig. S2 ). In view of the fact that tricyclazole has greater affinity for 3HNR than for 4HNR [14] , these observations could only be rationalized by assuming that dalesconols A ( 1 ) and B ( 2 ) were constructed by combinations of two DHN units with 3HN and 4HN motifs, respectively ( Fig. 1b ), whereas dalesconol C ( 3 ) was produced by the sequential coupling of three 3HN moieties ( Fig. 1c ). Moreover, that dalesconols A and B shared the same starting unit (DHN) with DHN–melanin was reinforced by the edge-cutting difference in the darkness (signifying the pigment formation) of the matured mycelia of D. eschscholzii cultured with and without the tricyclazole exposure ( Supplementary Fig. S3 ; the residual colour could be due to the otherwise produced fungal pigment(s)). 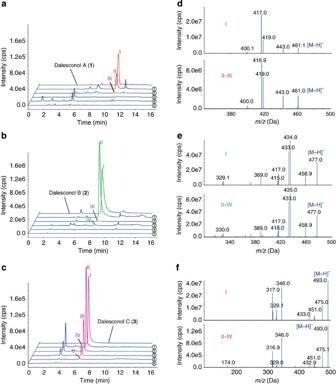Figure 3: LC–MS/MS screenings for dalesconols A–C (1–3) from tricyclazole-exposed fungal cultures. The samples were prepared from the EtOAc extracts ofD. eschscholziicultures without (1) and with exposures to tricyclazole at 30 (2), 50 (3), 100 (4) and 150 mg l−1(5). The LC–MS/MS profiles in an EIC mode (a–c) were acquired in MRM (multiple reaction monitoring) mode where the authentic dalesconols A–C signified in the ESI (electrospray ionization interface) /MS/MS product ion spectrum (d–f). Figure 3: LC–MS/MS screenings for dalesconols A–C (1–3) from tricyclazole-exposed fungal cultures. The samples were prepared from the EtOAc extracts of D. eschscholzii cultures without (1) and with exposures to tricyclazole at 30 (2), 50 (3), 100 (4) and 150 mg l −1 (5). The LC–MS/MS profiles in an EIC mode ( a – c ) were acquired in MRM (multiple reaction monitoring) mode where the authentic dalesconols A–C signified in the ESI (electrospray ionization interface) /MS/MS product ion spectrum ( d – f ). Full size image Involvement of laccase in generating naphthol radicals Following the tricyclazole exposure test, we investigated the mechanism by which these naphthol residues combine covalently to form polyketides 1 – 3 . As their (+)- and (−)-enantiomers are both produced, we proposed that the DHN, 3HN and 4HN motifs could form C – C bonds via either radical or cationic intermediates with sp 2 -hybridized reactive carbon centres without assured stereoselectivity. Correlating to the capability of a fungal laccase catalyzing the coupling reaction of phenolic molecules [16] , we hypothesized that the fungus could have produced laccase(s) capable of catalyzing the C – C bondage among naphthol motifs to give the corresponding enantiomeric mixtures. Using the protocol detailed elsewhere [17] , the presence of laccase in the fungal protein was ensured by the non-denaturing polyacrylamide gel electrophoresis (PAGE) analysis utilizing the substrate ABTS (2,2′-azinobis-(3-ethylbenzthiazoline-6-sulphonate)), which gave characteristically the green band upon the oxidation catalyzed by the enzyme ( Supplementary Fig. S4 ). To our expectation, a laccase-coding gene lacTL was found as a downstream gene in the pksTL gene cluster of the fungal strain (GenBank Nucleotide Core accession code: JX025148 ) by genome mining, and the knockout of the gene deprived the fungus of its productivity of polyketides 1 – 3 and dihydrosphaerolone ( Fig. 2b ; Supplementary Fig. S5 ), indicating that, in consortium with the aforementioned pksTL , this gene participates in the construction of the dalesconol framework from naphthol-based starter molecules ( Fig. 2a ). To confirm the involvement of naphthol radicals in the biosynthesis of 1 – 3 , the electron spin resonance (ESR) was applied to detect the presence of DHN radical generated upon the exposure of the naphthol to the fungal cellular proteins ( Fig. 4 ). The participation of the radical in constructing dalesconols A–C ( 1 – 3 ) was further reinforced by the free radical-scavenging experimentation. The fungus was cultured separately with exposures to an inorganic (MgSO 4 at 2.5 g l −1 ) and two organic (vitamins C and E, both at 30 mg l −1 ) free radical scavengers [18] , [19] . After 8-day cultivation, the culture broths were harvested, and their EtOAc extracts were analyzed by the LC–MS/MS method, indicating that the addition of MgSO 4 and vitamin C inhibited the production of dalesconols A–C ( 1 – 3 ). However, the addition of vitamin E did not show such an effect ( Supplementary Fig. S6 ). 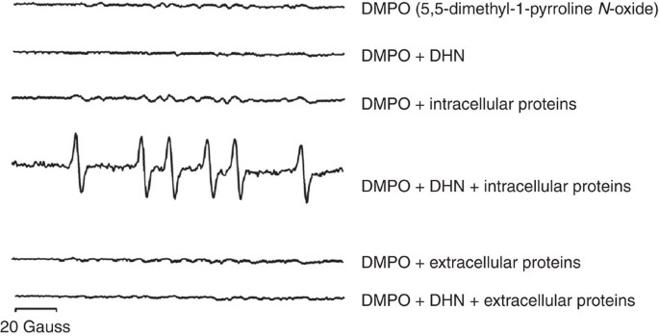Figure 4: ESR spectral detection of DHN radical generated in the presence of the fungal intracellular proteins. DMPO was used as a radical stabilizer to facilitate the measurement. Figure 4: ESR spectral detection of DHN radical generated in the presence of the fungal intracellular proteins. DMPO was used as a radical stabilizer to facilitate the measurement. Full size image Probing the (−)-e.e. in the fungal production of dalesconols With the coupling pattern of naphthol radicals addressed above, we were passionate about the determinant for the (−)-e.e. of dalesconols A–C ( 1 – 3 ). Owing to the close similarity in biosynthetic pathways of the three polyketides ( Fig. 1 ), our subsequent attention was focused on the formation process of dalesconol A ( 1 ). Inspired by the aforementioned biosynthetic information, we tested for the enzymatic transformability of the naphthol precursor into the desired di- and trimer ( Fig. 1b,c ), but failed most likely because of the extraordinary reactivity of the short-lived radicals, for which DMPO (5,5-dimethyl-1-pyrroline- N -oxide) had to be used as a stabilizer to facilitate the ESR measurement of radicals in this work ( Fig. 4 ) and elsewhere [20] . It is neither advisable to feed acylated naphthol dimers as pro-substrates for the tandem catalyses of lipases and laccases because of the enantio-complementary property of the former [21] . However, a scrutiny for the prochirality suggested that the discerned e.e. could be due to the conformational dominance of naphthol dimer radicals with a particular helicity. This hypothesis was reasoned as well by the X-ray crystal structure of (−)- and (+)-daeschol A (the immediate precursor of dalesconol A 6 ) with the dihedral angle γ C1−C2−C3−C4 (hereafter referred to as 'γ') of +72.5° and −72.5° ( Supplementary Fig. S7 ), signifying the different conformers of the naphthol dimer radical d ( Fig. 5 ). Subsequently, the molecular dynamics (MD) and quantum mechanical (QM) calculations were both performed to compare theoretically the conformational preference of radical d as a ligand of the ascomycete laccase (Protein Data Bank (PDB) accession code: 3QPK ) [22] , [23] , which was selected for the study in view of its homology to LacTL, and the high structural conservation in the active site of the existing microbial laccases [24] . Thus, two independent 1-ns MD simulations were carried out starting from positively and negatively angled naphthol dimer radicals, whose interchangeability could be supposed to be prohibited by the high energy barrier ( Supplementary Fig. S8 ). As a ligand of 3QPK, radical d was computed to have three typical conformations with γ values of +103.0±15.8°, +68.4±12.6° and −61.5±8.9° ( Fig. 5 ). Correspondingly, the three lowest energy conformers in the MD simulations, d - 1 ( γ =+99.4°), d - 2 ( γ =+57.9°) and d-3 ( γ =−63.1°), were abstracted to investigate their interaction patterns with the laccase ( Fig. 6 ). The O and H atoms in the hydroxyl and carbonyl groups of d conformers were involved in the intermolecular hydrogen bonding with the O···H distances being about 2.27 ( d - 1 ), 2.31 ( d - 2 ) and 2.35 Å ( d - 3 ), respectively. In 'laccase··· d - 1 ' and 'laccase··· d - 2 ' complexes, π–π stackings were discerned between the naphthol rings and the aromatic moiety of Phe427 ( Fig. 6a,b ). The QM calculations at B3LYP/6–31G(d) level with small models (consisting of d and its local interacting residues) demonstrated that d-1 was more stable than d-3 as the latter had an extra relative energy of 0.53 kcal mol −1 over the former. This results highlighted that the conformers (such as d-1 and d-2 ) in favour of generating (–)-daeschol A were at least twice more than those (represented by d-3 ) allowing the production of (+)-daeschol A ( Supplementary Fig. S9 ). 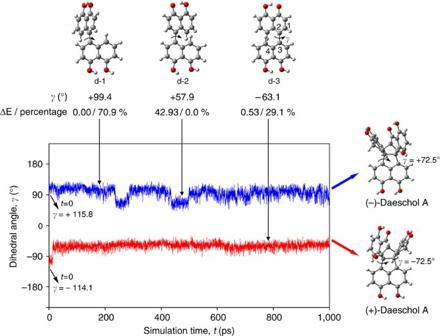Figure 5: Evolution of dihedral angleγC1−C2−C3−C4(°) in the naphthol dimer radical (d) along the simulation time. Starting fromdconfigurations with positive (blue) and negative (red) dihedral angles, two independent MD simulations are carried out in the canonical (constantN,V,T) ensemble within AmberFF03 framework. Relative energy (ΔE) is in kcal mol−1. Figure 5: Evolution of dihedral angle γ C1−C2−C3−C4 (°) in the naphthol dimer radical (d) along the simulation time. Starting from d configurations with positive (blue) and negative (red) dihedral angles, two independent MD simulations are carried out in the canonical (constant N , V , T ) ensemble within AmberFF03 framework. Relative energy (ΔE) is in kcal mol −1 . 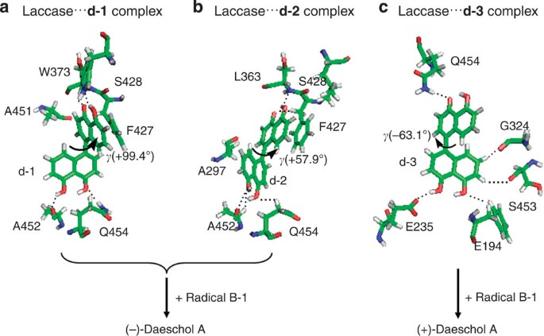Figure 6: Computed interactions between ascomycete laccase and naphthol dimer radical (d). The conformations with different dihedral angles are represented by: (a)d-1, (b)d-2and (c)d-3. Full size image Figure 6: Computed interactions between ascomycete laccase and naphthol dimer radical (d). The conformations with different dihedral angles are represented by: ( a ) d-1 , ( b ) d-2 and ( c ) d-3 . Full size image Because of the central significance, the formation of C–C bonds has appeared as a common research topic in both organic synthesis [25] and synthetic biology [2] . Nature's trick in constructing C–C covalent bonds seems more versatile and unforeseeable, but remains poorly understood as persuaded by a glance at the complex structures of the fungal metabolites 1 – 3 , and of the phytochemical-based anticancer drug taxol. The present investigation has disclosed that the promiscuous and atropselective couplings of naphthol radicals afford the unique structural feature and e.e. of dalesconols under a consortium of genes in different gene clusters of D. eschscholzii . To our knowledge, this is the first report dealing with a fungal synthesis of bioactive polyketides via C–C bond formations among hydroxynaphthalene motifs. Naphthol starters were hypothesized as the building blocks by inspecting the aromatization and oxygenation patterns of dalesconols A–C ( 1 – 3 ). This proposal was supported by a genome-mining approach that led to the identification of pksTL involved in the assembly of 4HN starter, and the 4HNR- and 3HNR-encoding genes located in different gene clusters of the fungus. The genetic information was in agreement with the inhibition test using tricyclazole, which was reported to modulate the fungal generation of 3HN and DHN from 4HN through differentiated inhibitions of 3HNR and 4HNR [14] . As screened by the LC–MS/MS analysis, the fungal exposure to tricyclazole attenuated (at 30 and 50 mg l −1 ) or abolished (at 100 mg l −1 ) the production of 1 and 2 , indicating that DHN is solely the common starter molecule for both polyketides. However, dalesconol C ( 3 ) was still producible during those treatments with tricyclazole below 100 mg l −1 . Moreover, none of the polyketides 1 – 3 could be found in the fungal culture if exposed to tricyclazole at 150 mg l −1 ( Fig. 3 ). This obervation highlighted that compound 3 was biosynthesized from 3HN only, and confirmed that tricyclazole has greater affinity for 3HNR than for 4HNR [14] . Thus, the experimentation demonstrated that dalesconols A ( 1 ) and B ( 2 ) were constructed by combinations of two DHN units with 3HN and 4HN motifs, respectively, whereas dalesconol C ( 3 ) was produced by the sequential couplings of three 3HN moieties ( Fig. 1b,c ). This was substantiated by our observation that the concentration of dihydrosphaerolone (derived from scytalone and 3HN [15] ) decreased as the tricyclazole concentration increased, and that the darkness (signifying the DHN–melanin pigment formation) of the matured mycelia of D. eschscholzii faded away with the fungal exposure to the increased amounts of the inhibitor although the residual colour due to the otherwise produced fungal pigment(s) is independent of the inhibition test with tricyclazole ( Supplementary Fig. S3 ). Regarding the coupling process of the naphthol starters, we anticipated that the formation of C – C bonds was accomplished via either radical or cationic intermediates, where the sp 2 -hybridized reactive carbon centres might have allowed the generation of both (+)- and (−)-enantiomers of 1 – 3 . The subsequent ESR measurement confirmed the production of DHN radical upon its exposure to the fungal cellular protein ( Fig. 4 ). In view of the laccase-catalyzed covalent bondage of phenolic molecules [16] , this observation was remindful of the involvement of the fungal laccase in the C – C bondage among naphthol precursors. We therefore ensured the production of such fungal laccase by non-denaturing PAGE analysis using ABTS as a substrate, which turned green upon the enzyme-catalyzed oxidation ( Supplementary Fig. S4 ) [17] . The genomic data ascertained a laccase-encoding gene lacTL existing at the directly downstream locus of pksTL (GenBank Nucleotide Core accession code: JX025148 ). To substantiate further the participation of radicals in constructing 1 – 3 , the free radical-scavenging experimentation was conducted by culturing for 8 days the fungus with respective exposures to an inorganic (MgSO 4 ) and two organic (vitamins C and E) free radical scavengers. As a result, MgSO 4 and vitamin C inhibited the production of 1 – 3 ( Supplementary Fig. S6 ). Concerning the mechanism, the deprival of dalesconols A–C production upon the fungal exposure to MgSO 4 could be ascribed to the radical-quenching activity of the salt, which was shown to be able to attenuate the radical-generating capacity of an array of enzymes such as nicotinamide–adenine dinucleotide phosphate oxidase [18] . As a non-phenolic radical-trapping antioxidant, vitamin C can react with radicals through multiple mechanisms [19] . However, vitamin E, which should have a similar function, did not affect substantially the generation of 1 – 3 in our test. This can be presumed to be because of its super lipophilicity that may prevent its contact with the radicals inside fungal cells. Following the aforementioned disclosure of the coupling pattern of naphthol radicals, the determinant for the (−)-e.e. of dalesconols A–C ( 1 – 3 ) attracted our attention. To avoid repetition, we examined the formation process of 1 , which is apparently similar to those of 2 and 3 ( Fig. 1 ). Although the enzymatic di- and trimerization of the naphthol starter failed, the X-ray crystal structure of daeschol A (yielding 1 upon autooxidation [6] ) with the opposite dihedral angles ( γ =+72.5° and −72.5°) for the two enantiomers ( Supplementary Fig. S7 ) suggested that the discerned e.e. could be due to the conformational dominance of naphthol dimer radicals with a particular helicity upon their interactions with the laccase. Considering that the active site of the described microbial laccases is highly conservative [24] , the well-documented laccase 3QPK [22] , [23] was selected for the subsequent theoretical study because of its ascomycete fungal origin and high homology to LacTL. Thus, the MD simulations and QM calculations were accomplished to ascertain the conformational preference of radical d ( Fig. 1b ) as a ligand of the selected laccase. Interacted with 3QPK, the three typical conformations of radical d were calculated to have the well differentiated dihedral angles ( γ =+103.0±15.8°, +68.4±12.6° and −61.5±8.9°) ( Fig. 5 ), and the corresponding lowest-energy conformers d - 1 ( γ =+99.4°), d - 2 ( γ =+57.9°) and d-3 ( γ =−63.1°) were adopted to explore their interactions with 3QPK ( Fig. 6 ). As a result, the clear π–π stackings between the naphthol rings and the aromatic motif of Phe427 were discerned in 'laccase··· d - 1 ' and 'laccase··· d - 2 ' complexes ( Fig. 6a,b ). Furthermore, the QM calculation at B3LYP/6–31G (d) level highlighted that d-3 has an extra relative energy of 0.53 kcal mol −1 over d-1 . This computation suggested that the conformers, represented by d-1 and d-2 that lead to the generation of (–)-daeschol A, are at least twice more than those symbolized by d-3, which yields (+)-daeschol A. It is noteworthy that the two naphthol dimer radicals d-1 and d-3 can give theoretically two pairs of enantiomers with (8 R ,19 R ,28 R ,29 S )-, (8 S ,19 S ,28 S ,29 R )-, (8 S ,19 R ,28 R ,29 R )- and (8 R ,19 S ,28 S ,29 S )-configurations, the latter two options being negligible because of the higher relative energies ( Supplementary Fig. S9 ). In summary, a combination of tricyclazole exposure tests, free radical-scavenging experiments, ESR determination, computation and whole-genome sequencing has demonstrated that the unusual framework and substitution pattern of dalesconols A–C ( 1 – 3 ) are generated, under a consortium of genes in different clusters, through the promiscuous and atropselective coupling of naphthol radicals derived from 4HN, 3HN and DHN. The (−)-e.e. discerned with these polyketides was theoretically predicted to be due to the laccase-favored conformational dominance of the naphthol dimer radical with its helicity leading to the fungal synthesis of the (−)-stereoisomer. The coupling promiscuity of naphthol radicals in the fungus, and the e.e. ascertained with dalesconols A–C are entirely unprecedented. The work highlights the possibility of increasing the structural diversity of secondary metabolites through radical couplings of phenolic precursors such as polyhydroxy naphthols that have been found in many fungi [14] , [15] and bacteria [4] . The findings are valuable for fertilizing or rethinking the concept and/or approach for the (bio)organic syntheses of important compounds from hydroxyphenylated starter molecules [7] , [26] , [27] , [28] . Furthermore, the investigation foretells as well that the laccase-catalyzed radical coupling among different starting phenols to form useful natural products of high complexity may be quite common. Our data update the existing views regarding the C–C bond formation via phenoxy radical couplings, and renewed knowledge about the construction logic of hydroxylnaphthalene starters produced by a broad taxonomic range of microbes [4] , [5] , [6] , [9] , [15] , [29] , [30] , which is overall of general importance in manipulating the microbial production and/or chemical synthesis of the immunosuppressants dalesconols A and B as well as other structurally related compounds of industrial potentials. Microbial and biochemical experiments D. eschscholzii obtained from the T. aridifolia gut was grown on ME agar medium containing in each liter ME (20 g), sucrose (20 g), peptone (1 g), agar (20 g) and appropriate volume of water. The fresh mycelia of the fungus were inoculated into 500 ml flasks, each of which was preloaded with 100 ml of ME medium (free of agar), followed by incubation for 8 days at 28 °C with an agitation of 120 r.p.m. DNA extraction, cellular protein extraction, enzyme assay and non-denaturing PAGE were completed and analyzed as described in the Supplementary Methods ( Supplementary Table S2; Supplementary Fig. S4 ). LC–MS/MS analysis The LC-MS/MS measurements was accomplished on an Agilent 1290 LC system (Agilent Technologies, Germany) hyphened with an AB SCIEX TRIPLE quadrupole 5500 mass spectrometer (AB SCIEX, Concord, Ontario, USA) with an Agilent ZORBAX SB-C18 column (5 μm, 150×2.1 mm), but for better resolutions using differentiated mobile phases including 4 mM ammonium formate containing a gradually increased amount of methanol (40–90% within 20 min, and kept at 90% for 5 min more) for the tricyclazole exposure and free radical-scavenging experiments, and 10 mM ammonium formate containing a gradually increased amount of acetonitrile (30→80% within 17 min) for the profile comparisons of the wild-type strain with the pksTL / lacTL gene knockout mutants. The electrospray ionization interface was operated in negative mode with the source temperature at 350 °C, curtain gas flowed at 20 l min −1 , and IonSpray voltage at −4500 V. The multiple reaction monitoring channels were monitored in windows covering the eluted compounds of interest (parent >daughter): electrospray ionization interface negative, dwell time 50 ms. Specifically, dalesconol A ( 1 ): 461.0>443.0 (collision energy (CE)-40; declustering potential (DP)-60), 461.0>417.0 (CE-52; DP-60); dalesconol B ( 2 ): 477.0>435.0 (CE-42; DP-50), 477.0>459.0 (CE-41; DP-50), 477.0>433.0 (CE-52; DP-50); dalesconol C ( 3 ): 493.0>346 (CE-100; DP-38), 493.0>475.0 (CE-38; DP-100), 493.0>317.0 (CE-52; DP-100). The samples and authentic materials were analyzed identically with the results retrieved from the main parent and daughter ion pair, and other ion pairs. All authentic samples used for the purpose were isolated in Tan's lab as described [5] , [6] . The filtrate of the fermented cultures was extracted exhaustively with ethyl acetate. In vacuo evaporation of solvent from each extract gave a brown oily residue, which was dissolved in MeOH, sonicated and filtered through 0.45 μm membrane filter to afford the sample solutions for LC–MS analyses. Tricyclazole exposure test Tricyclazole was dissolved quantitatively in ethanol to give the stock solution, which was added to sterile molten media at 30, 50, 100 and 150 mg l −1 in Petri dishes and Erlenmeyer flasks. Ethanol of equal volume was added into the plates as the blank control. The extracts derived from the 8-day culture were submitted for the LC–MS/MS analysis (see above), whereas those in Petri dishes were examined for the production of the DHN–melanin signified by the darkness of the medium after the 8-day cultivation ( Supplementary Fig. S3 ). Free radical-scavenging test To the culture medium, MgSO 4 (2.5 g l −1 ) and vitamins C and E (both at 30 mg l −1 ) were added separately before the inoculation of the fungal strain. After the 8-day cultivation, the broth derived from each culture was extracted and analyzed by the LC–MS/MS method ( Supplementary Fig. S6 ). ESR spectral measurement The ESR measurements were accomplished independently with intra- and extracellular proteins in phosphate (50 mM, pH 7.4) and citric acid–disodium hydrogen phosphate buffers (pH 2.5), respectively. After freshly dissolved in MeOH, DHN was quickly allowed to react with the fungal proteins in an O 2 -free box full of N 2 with DMPO present as a radical stabilizer, and the ESR spectra were acquired on a Bruker EMX (X-Band) ESR spectrophotometer at the following parameters: frequency: 9.761 GHz; modulation amplitude: 2.0 Gauss; power: 19.970 mW; centre field: 3480.0 G; sweep width: 100.0 G; and sweep time: 83.88 s. Genome sequencing The complete genome sequencing of D. eschscholzii IFB-TL01 was performed with a whole-genome shotgun sequencing strategy and Illumina Genome Analyser sequencing technology. To construct the genomic libraries, inserts of 500 bp and 6 kb were obtained, and the paired-end short reads were assembled using SOAPdenovo ( http://soap.genomics.org.cn ) [31] , giving a 32-fold coverage of the genome. And 99.15% of the reads were mapped into 875 contigs, ordered and orientated within 98 scaffolds ( Supplementary Table S4 ). The total length of all contigs is 35.5 Mb, and that of the scaffolds 35.8 Mb (including estimated sizes for the gaps). Within the achieved D. eschscholzii genome, 10,821 genes were predicted with an average size of 1,673.64 bp. This Whole Genome Shotgun project has been deposited at DDBJ/EMBL/GenBank under the accession AKGB00000000 (BioProject ID: PRJNA157267). The version described in this paper is the first which was numbered AKGB01000000. pksTL cloning and disruption of pksTL gene in D. eschscholzii Degenerate primers as listed in Supplementary Table S1 were designed according to the conserved regions of 4HN synthase, which have been possessed by other fungal strains such as Nodulisporium sp. ATCC74245 (AAD38786), Aspergillus terreus (BAB88689), A. fumigatus (AAC39471), Xylaria sp. BCC 1067 (AAM93545) and Colletotrichum lagenarium (BAA18956). The pksTL gene was obtained with degenerate and special primers by the genome-walking approach. A 1.0 kb Bam HI- Hind III fragment internal to the pksTL gene was amplified by PCR using TLU and TLL as primers and genome DNA as template, and then cloned into the vector pSH75 containing a hygromycin-resistant hph gene as a selectable marker between the A. nidulans PtrpC promoter and TtrpC terminator to produce pSHGDPKS. Fungal transformation was performed using restriction enzyme-mediated integration method as described [32] . Knockout of lacTL gene in D. eschscholzii D. eschscholzii was grown on potato dextrose agar plates for 10 days at 28 °C. Spores were collected, and the protoplasts were prepared with glucanex treatment. The 1015-bp fragment upstream of lacTL was amplified from D. eschscholzii by PCR using up-F and up-R as primers. The obtained fragment was digested with Bgl α/ EcoR δ, and inserted into vector pSH75 digested with the same restriction enzymes to give pLAC1. The 902-bp fragment downstream of lacTL was amplified using down-F and down-R as primers, digested with Bam H − / Hin dβ, and ligated into pLAC1 to produce the disruption vector pLAC2. The knockout cassette including a selection mark gene hph was amplified from pLAC2, and transformed into D. eschscholzii as described [32] . The mutant strains were identified by diagnostic PCR using both external and internal primes ( Supplementary Fig. S5 ). All the gene-specific primes used in this work were listed in Supplementary Table S1 . Force field parameterization for ligands The force field parameters of ligands (including naphthol radical bicopolymer d and daeschol A) were derived by the QM calculation with the Gaussian 09 program [33] . Hartree–Fock method at 6-31G** level was employed to optimize the geometries of these molecules in gas phase. Then, single-point calculations were carried out using the B3LYP method with cc-pVTZ basis set. The IEFPCM continuum solvent model was applied to mimic an organic solvent environment ( ε =4) [34] . The partial charges of the drug molecules were derived by fitting to electrostatic potential using the restrained ESP method [35] , [36] , [37] . MD simulations The X-ray crystal structure of the laccase with a PDB code of 3QPK [22] , [23] was taken as the starting structure to investigate the conformational diversities of naphthol dimer radical d and daeschol A ( Fig. 1 ) in the presence of laccase. The complex was solvated in a periodic TIP3P box with about 4282 water molecules. The minimum distance from the protein atom to the edge of the box was set to be about 10.0 Å, and 59 sodium counterion was added to neutralize the charge. A cutoff radius of 12.5 Å was applied for van der Waals and electrostatic interactions. The particle-mesh Ewald method [38] was used for evaluation of the long-range electrostatic interactions. To relax the initial structures, two-step energy minimizations were performed: (i) 15,000 steps of steeped descent followed by 10,000 conjugate gradient minimization, with a 500 kcal mol −1 restraint force on the protein molecule; (ii) 15,000 steps of steeped descent followed by 10,000 steps of conjugate gradient minimization with no restraints. The system was then heated from 0 to 300 K over 500 ps with harmonic constraints on protein, and a 1-ns MD simulation was performed in the NVT [standing respectively for constant numbers of atoms (N), volume (V) and temperature (T)] ensemble with a time step of 2 fs. The temperature was kept constant using the Berendsen temperature algorithm [39] . The SHAKE algorithm [40] was employed to constrain all bonds involving hydrogen atoms. All the energy minimization and MD simulation were carried out with the FF03 force field [34] in AMBER 9 program [41] . Relative energy calculations On the basis of the simulated complexes, the lowest-energy conformations along the MD trajectories were taken out to investigate the relative energies of various conformers (either for naphthol dimer radical d or daeschol A) interacted with laccase. It was difficult to perform conventional QM calculations on large-sized proteins. So, the binding domains with several residues were employed. All the energy calculations were carried out at B3LYP/6–31G level. How to cite this article: Fang, W. et al . Naphthol radical couplings determine structural features and enantiomeric excess of dalesconols in Daldinia eschscholzii . Nat. Commun. 3:1039 doi: 10.1038/ncomms2031 (2012).